Ultra-sensitive optical oxygen sensors for characterization of nearly anoxic systems Oxygen quantification in trace amounts is essential in many fields of science and technology. Optical oxygen sensors proved invaluable tools for oxygen measurements in a broad concentration range, but until now neither optical nor electrochemical oxygen sensors were able to quantify oxygen in the sub-nanomolar concentration range. Herein we present new optical oxygen-sensing materials with unmatched sensitivity. They rely on the combination of ultra-long decaying (several 100 ms lifetime) phosphorescent boron- and aluminium-chelates, and highly oxygen-permeable and chemically stable perfluorinated polymers. The sensitivity of the new sensors is improved up to 20-fold compared with state-of-the-art analogues. The limits of detection are as low as 5 p.p.b., volume in gas phase under atmospheric pressure or 7 pM in solution. The sensors enable completely new applications for monitoring of oxygen in previously inaccessible concentration ranges. Oxygen undoubtedly belongs to the most important analytes on earth. Traditionally, most oxygen sensors were designed for the physiological range. However, numerous applications require monitoring of oxygen at significantly lower concentrations, for example, corrosion protection [1] , surface treatment [2] , the semiconductor industry [3] and biological research. For instance, it was demonstrated that bacteria can show respiration and potentially aerobic growth far below the Pasteur point (~10 μM dissolved oxygen (DO)) [4] , [5] , [6] . Recently, sensors that quantify DO in concentration ranges of 100 nM and below have gained special interest as biologists explore aerobic life in areas very close to anoxic conditions [7] . Unfortunately, few sensors are capable to resolve at such low concentration [8] , [9] , and measurements below 0.5 nM are currently impossible. Optical sensors proved to be indispensable tools for oxygen quantification that have mostly replaced the more conventional Clark electrode. Their advantages include minimal invasiveness, simplicity, suitability for miniaturization, versatility of formats (planar optodes, fibre-optic sensors, micro- and nanoparticles, paints and so on) and suitability for imaging of oxygen distribution on surfaces or in volume. Moreover, optical oxygen sensors are tuneable over a wide range of concentrations. Optical oxygen sensors rely on quenching of a phosphorescent indicator by the analyte. Both the nature of the indicator and the matrix (which acts as a solvent and support for the dye and as a permeation-selective barrier) are of great importance since the sensitivity of an oxygen sensor is roughly proportional to the luminescence decay time of the indicator and to the oxygen permeability of the matrix [10] . State-of-the-art indicators are dominated by phosphorescent complexes with platinum group metals that possess decay times varying from microseconds to a few milliseconds [11] , [12] , [13] , [14] . Dyes with significantly longer decay times are extremely rare and are so far limited to fullerenes [9] , [15] (which have rather low luminescence brightness at ambient temperatures) and some phosphorescent BF 2 -chelates [16] , [17] , [18] , [19] . Both classes are not inherently compatible with highly oxygen-permeable matrices (for example, silicone and Teflon AF). Hence, the sensors based on these indicators and other matrices (for example, ethylcellulose and polystyrene (PS)) [9] are not drastically more sensitive than sensors relying on more conventional dyes (for example, Pd(II) porphyrins) immobilized in highly oxygen-permeable polymers [20] . Herein, we present a new type of oxygen-sensing materials that show sensitivities well beyond state-of-the-art trace oxygen sensors. They rely on new blue light-excitable BF 2 and Al(III) chelates featuring ultra-long room temperature phosphorescence. The chelates are modified with perfluoroalkyl chains to ensure compatibility with highly oxygen-permeable and chemically inert perfluorinated polymers. The resulted ultra-sensitive sensors are ideally suitable for characterization of nearly anoxic systems. Photophysical properties The new-sensing materials rely on novel difluoroboron- and aluminium chelates of 9-hydroxyphenalenone (HPhN; Fig. 1 ) [21] and its benzannelated derivative 6-hydroxybenz[de]anthracene-7-on (HBAN; scheme 1; ref. 22 ). In contrast to the common fluorescent difluoroboron chelates of dipyrromethenes and tetraarylazadipyrromethenes [23] , [24] , the new difluoroboron-based dyes simultaneously show prompt fluorescence, delayed fluorescence and phosphorescence when embedded in polymers ( Fig. 2a,b ). Room temperature phosphorescence is an extremely rare phenomenon for compounds with no heavy atoms. It was previously observed for BF 2 -chelates of aliphatic β-diketones coupled to polylactic acid [16] , [17] or physically entrapped in the same polymer [19] . This work and our results indicate that phosphorescence of aliphatic and aromatic BF 2 -chelates of β-diketones appears to be a general phenomenon. As can be seen, the extension of π-conjugation in HPhN derivatives results in bathochromic shifts of absorption, fluorescence and phosphorescence compared with the reported aliphatic diketonate chelates. In fact, the absorption of the HPhN and HBAN difluoroboron chelates peaks at 450 and 459 nm, respectively, ( ε 450 =10.2 × 10 3 M −1 cm −1 and ε 459 =12.9 × 10 3 M −1 cm −1 ). This enables excitation with bright blue 450 and 470 nm LEDs and with conventional white light sources. Temperature affects the quantum yields of all three emissions. As expected, the phosphorescence QYs decrease at higher temperature and the delayed fluorescence becomes stronger ( Fig. 2b ). Since both phosphorescence and delayed fluorescence possess virtually identical decay times ( Supplementary Fig. 1 ) and are quenched by oxygen to the same extent, their ratio can be used to eliminate temperature crosstalk. Importantly, prompt fluorescence is suitable for referencing purposes, as it is not affected by oxygen. However, the most outstanding property of these dyes is their extraordinary long phosphorescence decay time of 360 and 730 ms for BF 2 (HPhN) and BF 2 (HBAN), respectively (in PS at 20 °C), which, to the best of our knowledge, are the longest decay times recorded for visible light-excitable dyes. This is likely due to the rigid aromatic backbone structure of the dyes. 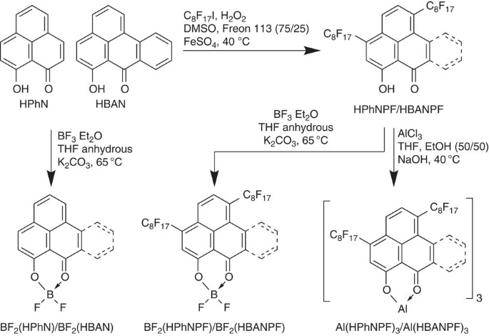Figure 1: Synthesis of the borondifluoride chelates and aluminium complexes. . Despite those long decay times, the phosphorescence quantum yields are fairly high ( Table 1 and Supplementary Table 1 ). Figure 1: Synthesis of the borondifluoride chelates and aluminium complexes. . 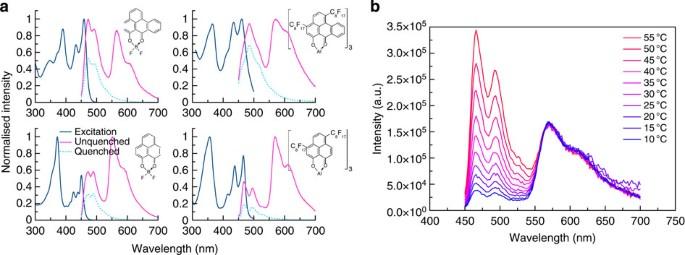Figure 2: Spectral properties of the oxygen indicators. (a) Excitation and emission spectra of HBAN and HPhN difluoroboron chelates in PS and aluminium complexes in Teflon AF 1600. (b) Temperature-dependent emission spectra of Al(HPhNPF)3in Hyflon AD 60 under deoxygenated conditions acquired with a delay of 0.5 ms after excitation. Full size image Figure 2: Spectral properties of the oxygen indicators. ( a ) Excitation and emission spectra of HBAN and HPhN difluoroboron chelates in PS and aluminium complexes in Teflon AF 1600. ( b ) Temperature-dependent emission spectra of Al(HPhNPF) 3 in Hyflon AD 60 under deoxygenated conditions acquired with a delay of 0.5 ms after excitation. Full size image Table 1 Photophysical and sensing properties of trace oxygen sensors at 20 °C. Full size table Ultra-sensitive oxygen-sensing materials Owing to the exceptionally long lifetimes of these chelates, resulting sensing materials are expected to have sensitivities orders of magnitude above those based on conventional sensing chemistries. Indeed, sensors composed of difluoroboron chelates in PS show very high sensitivities, even though PS has only moderate oxygen permeability ( P ≈8.8 × 10 −16 mol m −1 s −1 Pa −1 ; ref. 25 ) K SV for BF 2 (HPhN)- and BF 2 (HBAN)-based sensors was 60 × 10 −3 and 120 × 10 −3 p.p.m. v. −1 , respectively, ( Fig. 3a ), which makes them suitable for monitoring sub-nanomolar DO concentrations. The limit of detection for the BF 2 (HBAN)-based material, assuming a resolution of 0.5% I 0 , is in fact 45 p.p.b.v. (gas phase) or 60 pM (DO). Both sensing materials surpass the sensitivity of nearly all previously published sensors. Still, highly permeable matrices such as Hyflon, Teflon AF and poly(trimethylsilylpropyne) can potentially be used to create even more sensitive materials. Poly(trimethylsilylpropyne) has the highest known oxygen permeability ( P ≈23,000 × 10 −16 mol m −1 s −1 Pa −1 ; ref. 26 ) but was not considered because of poor chemical stability and possession of double bonds that are prone to oxidation and thus analyte consumption [27] , [28] . Hyflon and Teflon AF are amorphous, glassy, perfluorinated copolymers that combine high free volume and unmatched chemical stability. In this work we used Hyflon AD 60 ( P ≈170 × 10 −16 mol m −1 s −1 Pa −1 ; ref. 29 ) and Teflon AF 1600 ( P ≈1,200 × 10 −16 mol m −1 s −1 Pa −1 ; ref. 30 ). Unfortunately, most conventional dyes, as well as BF 2 (HPhN) and BF 2 (HBAN), show extremely poor solubility in these matrices and aggregate readily. We failed to obtain usable sensors based on the BF 2 -chelates due to poor luminescence in perfluorinated polymers at any relevant concentration (0.01–1% wt. of the dyes in respect to the polymer). Therefore, in order to render the indicators soluble in Hyflon and Teflon AF, HPhN and HBAN were perfluoroalkylated with perfluorooctyl iodide (scheme 1). The resulting ligands 9-hydroxy-4,7-diperfluorooctyl-1H-phenalenone (HPhNPF) and 6-hydroxy-1,4-diperfluorooctyl-7H-benzo[de]anthracen-7-one (HBANPF) bear two C 8 F 17 chains each, although in the case of HBANPF there is some impurity of tri-substituted ligand ( Supplementary Figs 2 and 3 ). As indicated by nuclear Overhauser effect spectroscopy (NOESY) and heteronuclear multiple-bond correlation spectroscopy (HMBC) spectra ( Supplementary Figs 4 and 5 ), a single isomer appears to be the predominant product for HPhNPF ( Supplementary Fig. 6 ). The 1 H nuclear magnetic resonance (NMR) and correlation spectroscopy (COSY) spectra for HBANPF ( Supplementary Figs 7 and 8 ) showed no significant substitution in the benzannelated ring. Complete separation of the tri-substituted derivate is very challenging owing to the very high similarity; however, both tri- and disubstituted derivates are expected to have very similar photophysical properties und solubility. It was found that perfluoroalkylated derivates of the difluoroboron chelates have low chemical stability and dissociate in solution in presence of traces of water ( Supplementary Fig. 9 ). Hence, aluminium complexes (Al(HPhNPF) 3 and Al(HBANPF) 3 ; scheme 1) were prepared in an attempt to obtain more stable indicators. Indeed, dissociation was not observed for the aluminium chelates and they dissolve readily in fluorinated solvents (octafluorotoluene and perfluorodecalin) and also in Hyflon and Teflon AF. Owing to the octahedral structure of the Al(III) complexes and unsymmetric substitution pattern of the ligands four sterioisomers are possible, which are inseparable because of their extreme similarity. The photophysical properties of the isomers are expected to be virtually identical. Similar to the BF 2 -chelates, the Al(III) complexes possess prompt fluorescence, delayed fluorescence and phosphorescence ( Fig. 1 ). The phosphorescence decay times (250 ms for Al(HPhNPF) 3 and 350 ms for Al(HBANPF) 3 at 20 °C in Teflon AF 1600) are slightly shorter than those of the BF 2 -chelates, and the Al(III) complexes possess higher molar absorption coefficients ( ε 465 =23.2 × 10 3 M −1 cm −1 and ε 459 =27.1 × 10 3 M −1 cm −1 for Al(HPhNPF) 3 and Al(HBANPF) 3 , respectively). The oxygen-sensing materials based on these Al(III) complexes embedded in Hyflon show extremely high sensitivities ( Fig. 3b ). In fact, the K SV values are as high as 590 × 10 −3 p.p.m. v. −1 (for Al(HBANPF) 3 , Table 1 ) and the sensors resolve up to 10 p.p.b.v. or 12 pM DO. They are about one order of magnitude more sensitive than the state-of-the-art sensors based on fullerenes ( Table 1 ) [14] . The sensors based on Teflon AF 1600 show a twofold increase in sensitivity compared with the Hyflon-based ones. Al(HBANPF) 3 in Teflon AF 1600 is the most sensitive sensor material presented, with a K SV of 960 × 10 −3 p.p.m. v. −1 and a detection limit of 5 p.p.b.v. or 7 pM. Potentially, even more sensitive sensor materials based on Teflon AF 2400 ( P ≈3000 × 10 −16 mol m −1 s −1 Pa −1 ; ref. 30 ) showed signs of aggregation and were therefore not further investigated. Importantly, the Stern–Volmer plots for the phosphorescence decay time are similar to those obtained for the intensity measurements ( Fig. 3b and Supplementary Fig. 10 ) so both read-out schemes (ratiometric intensity or decay time) can be used. It should be mentioned that sensitivities are so high that obtaining reliable calibrations becomes rather challenging. Even high-purity nitrogen contains oxygen impurities in the low p.p.m. range, hence all aluminium complex-based sensor materials were calibrated using a standard addition method described in the experimental section. 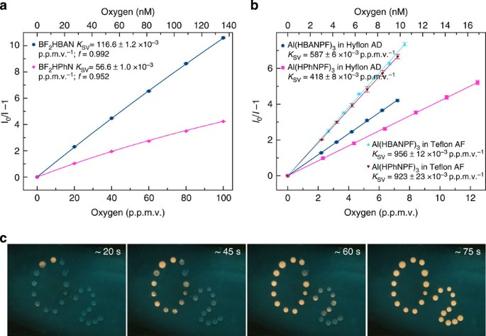Figure 3: Oxygen sensitivity of the trace sensors at 20 °C. (a) Stern–Volmer plots for BF2HBAN and BF2HPhN in PS. (b) Stern–Volmer plots for the aluminium complexes. (c) Photographic images of the Al(HPhNPF)3/Hyflon AD 60 sensor under illumination with a 366-nm line of a ultraviolet lamp. Bluish prompt fluorescence remains constant, and the intense yellow phosphorescence slowly appears for the areas covered with anaerobic sodium sulphite solution (5% wt, containing traces of Co2+as a catalyst). Figure 3: Oxygen sensitivity of the trace sensors at 20 °C. ( a ) Stern–Volmer plots for BF 2 HBAN and BF 2 HPhN in PS. ( b ) Stern–Volmer plots for the aluminium complexes. ( c ) Photographic images of the Al(HPhNPF) 3 /Hyflon AD 60 sensor under illumination with a 366-nm line of a ultraviolet lamp. Bluish prompt fluorescence remains constant, and the intense yellow phosphorescence slowly appears for the areas covered with anaerobic sodium sulphite solution (5% wt, containing traces of Co 2+ as a catalyst). Full size image Temperature is known to affect the response of all optical sensors; thus the temperature dependence of the new sensors was investigated ( Supplementary Fig. 11 ). In contrast to most oxygen sensors, the Stern–Volmer constants K SV decrease at higher temperature. This can be explained by a relatively strong effect of temperature on the phosphorescence decay time τ 0 (280, 250 and 220 ms at 5, 20 and 35 °C, respectively, for Al(HPhNPF) 3 in Hyflon AD 60) and a negligible influence on the bimolecular quenching constant k q (1.65, 1.65 and 1.69 p.p.m. v. −1 ms −1 at 5, 20 and 35 °C, respectively). This indicates that in contrast to most polymers, the oxygen permeability of Hyflon AD 60 appears to be barely affected by temperature. Application example To illustrate potential applications of these trace oxygen sensors, the kinetics of oxygen consumption during enzymatic oxidation of glucose was monitored as it approached anoxic conditions ( Fig. 4 ). Aqueous solutions of glucose oxidase, catalase and glucose were combined in a closed stirred vessel, and the oxygen concentration was monitored with a set of sensors with overlapping ranges. In addition to the Al(HPhNPF) 3 /Hyflon sensor, two other oxygen sensors were used: a commercially available trace sensor from Pyroscience GmbH and a sensor based on Pd(II)-5,10,15,20-meso-tetrakis-(2,3,4,5,6-pentafluorphenyl)-porphyrin in Hyflon, which is comparable in sensitivity to previously published sensors [31] . 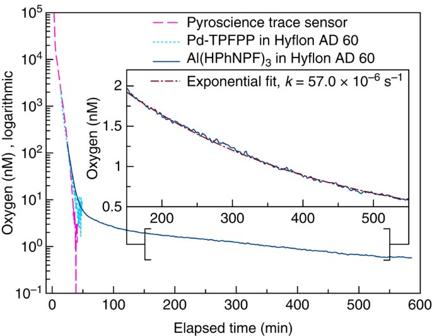Figure 4: Real-time monitoring of oxygen levels during enzymatic oxygen consumption. Three trace sensors with overlapping ranges are used to monitor oxidation of glucose catalysed by glucose oxidase. A running average of 3 data points was used for all sensors. Whereas, the reference sensors fail to resolve below 2–10 nM; the new ultra-trace sensor can reliably monitor oxygen even at much lower concentrations (insert). Figure 4 shows the high resolution of the new sensors in the ultra-trace region, whereas the other sensors fail to resolve oxygen concentrations below 1 nM. The insert shows a mono-exponential fit of the ultra-trace region corresponding to purely diffusion-controlled depletion of oxygen. Figure 4: Real-time monitoring of oxygen levels during enzymatic oxygen consumption. Three trace sensors with overlapping ranges are used to monitor oxidation of glucose catalysed by glucose oxidase. A running average of 3 data points was used for all sensors. Whereas, the reference sensors fail to resolve below 2–10 nM; the new ultra-trace sensor can reliably monitor oxygen even at much lower concentrations (insert). Full size image Precise quantification of oxygen impurity in inert gases represents another potential application of the new sensors. The Al(HPhNPF) 3 /Hyflon sensor was used to quantify oxygen content in high-purity gases obtained from Linde (Austria). For example, two samples of compressed nitrogen 5.0 (99.999%, <10 p.p.m.v. O 2 ) contained 3.7 and 2.5 p.p.m.v. O 2 , whereas compressed nitrogen 6.0 (99.9999%, <1 p.p.m.v. O 2 ) contained 0.52 p.p.m.v. O 2 , which is within the specifications of the gas manufacturer. We prepared new optical oxygen-sensing materials with unmatched sensitivity. The most sensitive shows an ~20-fold increase in sensitivity compared with state-of-the-art materials. Such extraordinary high-sensitivity results from the combination of extremely long phosphorescence decay times of the indicators and very high oxygen permeability of the matrix. Novel heavy metal-free chelates of rigid aromatic analogues of β-diketones represent unique indicators for oxygen sensors that feature absorption in the blue part of the electromagnetic spectrum, very long-decaying room temperature phosphorescence, good molar absorption coefficients and adequate quantum yields. The unique dual emission of the chelates (delayed fluorescence and phosphorescence) can be used for intrinsic temperature compensation. These sensors enable completely new applications for monitoring of oxygen in previously inaccessible concentration regions, and are likely to become invaluable tools in various fields of science and technology. Materials Nitrogen (99.9999% purity) and test gases (1,000 p.p.m.v. O 2 , rest N 2 ; and 20 p.p.m.v. O 2 , rest N 2 ) were obtained from Linde Gas (Austria; www.linde.at ), PS (molecular weight (MW) 250,000) and hydrogen peroxide (60%) were obtained from Fisher Scientific. Perfluorooctyl iodide and aquaphobe CF were bought from ABCR (Germany; www.abcr.de ). Teflon AF 1600 was acquired from DuPont (USA; www.dupont.com ). Hyflon AD 60 was obtained from Solvay (USA; www.solvayplastics.com ). Sodium sulphite was obtained from Carl Roth ( www.carlroth.com ). Boron trifluoride diethyl etherate, aluminium oxide (activated, neutral Brockmann I), aluminium(III) chloride, 1,1,2-trichloro-1,2,2-trifluoroethane (Freon 113), glucose oxidase from Aspergillus niger , catalase from bovine liver, anhydrous tetrahydrofuran (THF) and anhydrous dimethylsulphoxide were obtained from Aldrich, iron(II) sulphate heptahydrate from Merck, sodium hydroxide from Lactan (Austria; www.lactan.at ) and silicon E4 from Wacker (Germany; www.wacker.de ). Acetone and ethanol were acquired from Brenntag (Germany; www.brenntag.de ), and other solvents including the deuterated solvents were from VWR (Austria; www.at.vwr.com ). HPhN was obtained from Ramidus (Sweden; www.ramidus.se ) and HBAN was synthesized according to the literature procedure [22] . Synthesis of the BF 2 chelate of HPhN An amount of 294 mg (1.5 mmol) of HPhN were dissolved in 50 ml of anhydrous THF and 1.92 g (13.5 mmol) of boron trifluoride diethyl etherate were added. The solution was stirred for 1 h at 65 °C, the solvent was removed under vacuum and the product was purified on an aluminium oxide column using dichloromethane as an eluent. Yield: 300 mg (67%) of orange crystals. 1 H NMR (300 MHz, DMSO-d 6 , δ ): 8.94 (d, J =9.1 Hz, 2H), 8.70 (d, J =7.7 Hz, 2H), 8.03 (t, J =7.7 Hz, 1H), 7.62 ( d , J =9.1 Hz, 2H). Electron impact-direct injection-time of flight (EI-DI-TOF) ( m / z ): found 244.0499, calculated 244.0510. Synthesis of the BF 2 chelate of HBAN A quantity of 369 mg (1.5 mmol) of HBAN were dissolved in 60 ml of anhydrous THF, and 1.7 g (12 mmol) of boron trifluoride diethyl etherate were added. The solution was stirred at 65 °C for 2 h, and 69 mg (0.5 mmol) of potassium carbonate were added and the stirring was continued for 2 h. The solvent was removed under vacuum and the product was purified on an aluminium oxide column using dichloromethane as an eluent. Yield: 340 mg (77%) of orange crystals. 1 H NMR (300 MHz, DMSO-d 6 , δ ): 9.26 (d, J =7.7 Hz, 1H), 9.04 (d, J =8.3 Hz, 1H), 8.91 (d, J =9.2 Hz, 1H), 8.69 (d, J =8.2 Hz, 1H), 8.50 (d, J =7.6 Hz, 1H), 8.21 (t, J =8.3 Hz, 1H), 7.97 (dt, J =21.2, 7.6 Hz, 2H), 7.61 (d, J =9.1 Hz, 1H). EI-DI-TOF ( m / z ): found 294.0671, calculated 294.0667. Synthesis of HPhNPF HPhN (1 g, 5.1 mmol) and FeSO 4 7 H 2 O (2.5 g, 9.0 mmol) were dissolved in 120 ml dimethylsulfoxide (DMSO) and 40 ml 1,1,2-trichloro-1,2,2-trifluoroethane in a 200 ml Schlenk flask. The whole reaction was conducted under argon atmosphere. The solution was heated to 40 °C and perfluorooctyl iodide (3.4 ml, 7.03 g, 12.9 mmol) was added. 60% H 2 O 2 (1.4 ml, 1.67 g, 49 mmol) was added drop-wise over 5 min. The solution turned red and formed black foam. After 30 min, 20 ml 1,1,2-trichloro-1,2,2-trifluoroethane were added and the foam dissolved. One hour after the start of the reaction, a second portion perfluorooctyl iodide (3.4 ml, 7.03 g, 12.9 mmol) was added and 60% H 2 O 2 (1.4 ml, 1.67 g, 49 mmol) was added drop-wise over 5 min. The reaction was continued for 1 h, then the reaction mixture was cooled to room temperature, and the DMSO and 1,1,2-trichloro-1,2,2-trifluoroethane phases were separated. The 1,1,2-trichloro-1,2,2-trifluoroethane phase was washed three times with 36% hydrochloric acid, once with water, and was dried over Na 2 SO 4 . After removing the solvent, 9.3 g reddish-brown oil were obtained. The product was purified on a silica-gel column with hexane and toluene as eluents. Yield: 700 mg (13%). R F 0.57 with toluene. 1 H NMR (300 MHz, CDCl 3 +Freon 113 (1:1 v/v), δ ): 16.75 (s, 1H), 8.77 (s, 1H ), 8.15-8.00 (m, 2H), 7.86 (d, J =7.9 Hz, 2H), 7.24 (d, J =9.3 Hz, 2H). DI-EI ( m / z ): 1,031.98 found, 1,031.98 calculated. Synthesis of HBANPF HBANPF was prepared using the same procedure as HPhNPF, but with a fivefold excess of perfluorooctyl iodide, and the reaction mixture was stirred stirred for 2 h at 40 °C and then overnight at room temperature. Yield 500 mg (23%) starting from 0.5 g HBAN. R F 0.69 with hexane/toluene 2/1. 1 H NMR (300 MHz, CDCl 3 +Freon 113 (1:1 v/v), δ ): 17.01 (s, 1H), 8.94 (s, 1H), 8.79 (d, J =8.2 Hz, 1H), 8.71 (d, J =7.9 Hz, 1H), 8.52 (d, J =8.3 Hz, 1H), 8.03 (d, J =8.2 Hz, 1H), 7.89 (t, J =7.6 Hz, 1H), 7.73 (t, J =7.5 Hz, 1H). DI-EI ( m / z ): 1,081.99 found, 1,081.99 calculated. Synthesis of the aluminium complex of HPhNPF HPhNPF (100 mg, 0.097 mmol) was dissolved in 20 ml THF and 20 ml ethanol. NaOH (5.9 mg, 0.15 mmol) and AlCl 3 (3.9 mg, 29 μmol) were added and the reaction mixture was stirred for 2.5 h at 40 °C. Then the reaction was stopped the product was extracted with 1,1,2-trichloro-1,2,2-trifluoroethane and the organic phase was washed twice with water. The organic layer was dried over Na 2 SO 4 and evaporated in vacuum. Five millilitres THF were added to the raw product and the mixture was placed in the freezer for a few hours. The THF phase was removed and new THF was added. The product was washed seven times following this procedure. Yield: 68.4 mg (74%). 1 H NMR (300 MHz, CDCl 3 +Freon 113 (1:1 v/v), δ ): 8.87-8.55 (m, 3H), 8.15-7.84 (m, 6H), 7.84-7.54 (m, 3H), 7.42-7.04 (m, 3H); matrix assisted laser desorption ionisation (MALDI) ( m / z ): [M+Na] + : 3,142.93 found, 3,142.90 calculated. Synthesis of the aluminium complex of HBANPF Al (HBANPF) 3 was prepared and purified with the same procedure as Al(HPhNPF) 3 . Yield 19.5 mg (31%) starting from 80 mg HBANPF. 1 H NMR (300 MHz, CDCl 3 , δ ): 9.2-8.2 (m, 9.9H), 8.06 (s, 3H), 8.0-7.2 (m, 7.2H); MALDI ( m / z ): [MH]+: 3,271.11 found, 3,270.96 calculated, (MH(with one additional C 8 F 17 -group))+: 3,689.02 found, 3,688.92 calculated. Preparation of the PS-based sensing materials The sensor ‘cocktails’ contained the dyes (0.02% w/w in respect to the polymer), PS (5% w/w in respect to the solvent) and chloroform. These were knife-coated on a glass slide using a 175-μm spacer. The resulting thickness for the dried layer is estimated to be 6 μm. Preparation of the Hyflon AD 60-based sensing materials Before coating, the glass slides were rendered hydrophobic with aquaphobe CF. The dyes (0.05% w/w in respect to the polymer) and the polymer (6% w/w in respect to the solvent) were dissolved in octafluorotoluene. Knife-coating on the glass slides using a 175-μm spacer yielded a layer thickness of ~12 μm. After a second coating with a 275-μm spacer and evaporation of the solvent an ~31-μm-thick layer was obtained. Preparation of the Teflon AF 1600-based sensing materials The sensors were prepared analogously to those based on Hyflon, but a 5% w/w solution of the polymer in octafluorotoluene was used. The thickness of the sensing layer was estimated to be 24 μm. Measurements 1 H NMR spectra were recorded on a 300 MHz instrument (Bruker). NOESY and HMBC spectra were acquired on an INOVA 500 MHz NMR spectrometer (Varian). DMSO-d6 was used for HPhN and HBAN and the respective BF 2 chelates and a mixture of 1,1,2-trichloro-1,2,2-trifluoroethane and CDCl 3 (1:1, v/v) was used for perfluorinated ligands and the respective chelates. Electron impact (EI; 70 eV) and MALDI-TOF mass spectra were recorded on a Waters GCT Premier equipped with direct insertion (DI) and on a Micromass TofSpec 2E, respectively. Absorption spectra were acquired on a Cary 50 UV-VIS spectrophotometer from Varian and the emission spectra on a Fluorolog 3 fluorescence spectrometer from Horiba Scientific equipped with a R2658 photomultiplier from Hamamatsu. The absolute luminescence quantum yields were determined using an integrating sphere from Horiba. The luminescence decay times for the sensing materials were measured with the Fluorolog 3 spectrometer in kinetic acquisition mode. Calibrations were obtained using a temperature-controlled flow-through cell combined with a gas-mixing device from Voegtlin (Switzerland; www.red-y.com ), which was used to mix nitrogen with 0.1% O 2 test gas (for the boron chelates) and nitrogen with 20 p.p.m.v. O 2 test gas (for the aluminium complexes). Calibrations for the aluminium complexes were further corrected for impurities in the nitrogen gas using a standard addition method, by measuring decay times under nitrogen und in oxygen-free sodium sulphite solution. The measured intensities under nitrogen were multiplied with the lifetime ratio (nitrogen/oxygen-free) to obtain the actual value for I 0 . All calibration points were corrected by the obtained intrinsic oxygen contamination. For additional information on photophysical properties of the dyes, see Supplementary Figs 12–16 . For NMR and mass spectroscopy analysis of the compounds in this article, see Supplementary Figs 17–28 . How to cite this article: Lehner, P. et al . Ultra-sensitive optical oxygen sensors for characterization of nearly anoxic systems. Nat. Commun. 5:4460 doi: 10.1038/ncomms5460 (2014).